CYLD negatively regulates transforming growth factor-β-signalling via deubiquitinating Akt Lung injury, whether induced by infection or caustic chemicals, initiates a series of complex wound-healing responses. If uncontrolled, these responses may lead to fibrotic lung diseases and loss of function. Thus, resolution of lung injury must be tightly regulated. The key regulatory proteins required for tightly controlling the resolution of lung injury have yet to be identified. Here we show that loss of deubiquitinase CYLD led to the development of lung fibrosis in mice after infection with Streptococcus pneumoniae . CYLD inhibited transforming growth factor-β-signalling and prevented lung fibrosis by decreasing the stability of Smad3 in an E3 ligase carboxy terminus of Hsc70-interacting protein-dependent manner. Moreover, CYLD decreases Smad3 stability by deubiquitinating K63-polyubiquitinated Akt. Together, our results unveil a role for CYLD in tightly regulating the resolution of lung injury and preventing fibrosis by deubiquitinating Akt. These studies may help develop new therapeutic strategies for preventing lung fibrosis. Lung injury represents a major cause of morbidity and mortality worldwide. Injurious stimuli such as infectious agents and caustic chemicals initiate a complex and dynamic series of host wound-healing responses. During the early stage of severe Streptococcus pneumoniae infections, pneumolysin induces acute lung injury (ALI) and lethality. As a critical host response, type 1 plasminogen activator inhibitor (PAI-1) is upregulated by S. pneumoniae , which provides protection against ALI by preventing alveolar hemorrhage [1] . Appropriate host response such as upregulated PAI-1 production is thus critical for repairing injured lung tissue and restoring its function. However, if uncontrolled, excessive PAI-1 will have an adverse effect on tissue remodelling process via enhanced accumulation of extracellular matrix in tissues [2] , [3] , [4] , [5] , [6] , [7] , [8] , [9] . Thus, PAI-1 expression must be tightly and dynamically regulated during the entire host wound-healing process. We previously found that deubiquitinase CYLD has a critical role in preventing excessive production of PAI-1 by suppressing its p38 MAPK-dependent expression. However, during lethal S. pneumoniae infection, excessive release of pneumolysin caused severe lung injury, which overwhelms the protective effect of available PAI-1, thereby leading to lethality. Interestingly, CYLD deficiency in the Cyld-deficient mouse results in excessive production of PAI-1, thus providing efficient protection against lethality [1] . Therefore, our previous study demonstrates that CYLD is a critical negative regulator for host survival during early stage of infection as Cyld-deficient mice have a much higher survival rate compared with wild-type (WT) mice. Because uncontrolled and excessive wound-healing response such as excessive PAI-1 production could result in lung fibrosis [3] , we hypothesized that Cyld-deficient mice that survived lethal S. pneumoniae infection may develop lung fibrosis, and CYLD the may thus act as a key regulator for the wound-healing process during the late stage of bacterial infections. Here we show that CYLD acts as a critical negative regulator for injury-induced fibrotic response by inhibiting transforming growth factor-β (TGF-β)-signalling. We further show that CYLD inhibits TGF-β-signalling via decreasing the stability of Smad3 protein in a glycogen synthase kinase3-β (GSK3β)-Hsc70-interacting protein (CHIP)-dependent manner. Interestingly, CYLD decreases Smad3 stability by directly deubiquitinating K63-polyubiquitinated Akt. These studies may bring new insights into the novel role of CYLD in regulating fibrosis and may lead to the identification of new therapeutic targets for treating these diseases. CYLD is a key negative regulator for lung fibrosis To test our hypothesis, we first determined whether CYLD deficiency leads to the development of lung fibrosis in a mouse model of lung injury induced by S. pneumoniae infection. As shown in Fig. 1a , the majority of WT mice that survived ALI appeared fully recovered without significant pathological changes. In contrast, Cyld −/− mice exhibited marked fibrotic pathological changes as evaluated by performing H&E staining. Further, histological analysis with Trichrome staining demonstrated significant collagen deposition (stained blue) in lungs of S. pneumoniae -inoculated Cyld −/− mice but not in WT mice. Moreover, S. pneumoniae -inoculated lungs of Cyld −/− mice also exhibited a hyperfibrotic response, with increased expression of fibrogenic gene type I and type III collagens (COL1A2 and COL3A1), connective tissue growth factor (CTGF) and PAI-1 compared with WT mouse lung ( Fig. 1b ). Similar to the lethal dose of S. pneumoniae , a sub-lethal dose of S. pneumoniae still exhibited a fibrotic effect, and the fibrotic response was significantly enhanced in Cyld −/− mice compared with WT mice ( Supplementary Fig. S1a ). Thus, it is evident that, regardless of the severity of infection, CYLD has a critical role in tightly controlling the fibrotic response and preventing fibrosis. 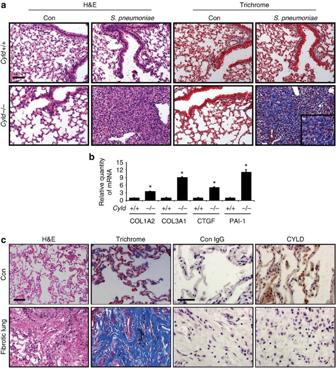Figure 1: CYLD is a negative regulator for lung fibrosis in mouse and human. (a) H&E and Masson's trichrome (Trichrome) staining of lung tissues fromCyld+/+andCyld−/−mice 2-weeks postS. pneumoniaeinfection (insert: ×400). Scale bars correspond to 200 μm. (b) Relative quantity of mRNA expression of type I and type III collagens (COL1A2 and COL3A1), CTGF and type 1 plasminogen activator inhibitor (PAI-1) compared with internal control Glyceraldehyde 3-phosphate dehydrogenase was measured in the lung tissues ofCyld+/+andCyld−/−mice 2-weeks postS. pneumoniaeinfection.*P<0.05 values are the means±s.d. (n=3). Un-paired Student'st-test was used for comparison withCyld+/+. (c) H&E, Masson's trichrome, and anti-CYLD staining of control (Con) and lung fibrosis tissues of human patients (Fibrotic lung). Lung fibrosis tissues were obtained from the patients with pulmonary fibrosis, during pneumonectomy, and normal control tissues were obtained from the patient with pneumothorax during the surgery. Slides are representative of 5 (Con) and 10 (Fibrotic) human lung tissues. Scale bars, 200 μm. Figure 1: CYLD is a negative regulator for lung fibrosis in mouse and human. ( a ) H&E and Masson's trichrome (Trichrome) staining of lung tissues from Cyld +/+ and Cyld −/− mice 2-weeks post S. pneumoniae infection (insert: ×400). Scale bars correspond to 200 μm. ( b ) Relative quantity of mRNA expression of type I and type III collagens (COL1A2 and COL3A1), CTGF and type 1 plasminogen activator inhibitor (PAI-1) compared with internal control Glyceraldehyde 3-phosphate dehydrogenase was measured in the lung tissues of Cyld +/+ and Cyld −/− mice 2-weeks post S. pneumoniae infection. *P< 0.05 values are the means±s.d. ( n =3). Un-paired Student's t -test was used for comparison with Cyld +/+ . ( c ) H&E, Masson's trichrome, and anti-CYLD staining of control (Con) and lung fibrosis tissues of human patients (Fibrotic lung). Lung fibrosis tissues were obtained from the patients with pulmonary fibrosis, during pneumonectomy, and normal control tissues were obtained from the patient with pneumothorax during the surgery. Slides are representative of 5 (Con) and 10 (Fibrotic) human lung tissues. Scale bars, 200 μm. Full size image On the basis that CYLD acts as a negative regulator for PAI-1 upregulation by inhibiting p38 MAPK-dependent PAI-1 expression [1] , we first determined whether CYLD inhibits S. pneumoniae -induced lung fibrosis also via inhibiting p38 MAPK signalling. Interestingly, treatment with p38-specific inhibitor SB203580 did not affect lung fibrosis in these Cyld −/− mice ( Supplementary Fig. S1b ). This unexpected finding thus led us to focus on determining a p38-independent molecular mechanism by which CYLD prevents development of lung fibrosis post-bacterial-infection. Among a number of signalling pathways involved in lung fibrosis, TGF-β-Smad signalling is crucial for regulating lung fibrosis, and S. pneumoniae has been shown to induce TGF-β-signalling [10] , [11] , [12] , [13] , [14] , [15] . Thus, we first determined whether S. pneumoniae induces TGF-β-expression. As shown in Supplementary Fig. S1c , S . pneumoniae induced TGF-β expression at late stage of infection when fibrosis develops, whereas it induced rapid p38 MAPK activation at early stage when lung injury is induced, followed by inactivation at late stage. These interesting results may well explain why inhibition of p38 using a specific inhibitor did not affect lung fibrosis in Cyld −/− mice and may also imply an important role of TGF-β-Smad in mediating S. pneumoniae -induced lung fibrosis. To further determine the clinical relevance of our finding in the mouse model, the expression level of CYLD protein in the lung of human patients with lung fibrosis was measured and compared with that in normal controls. As shown in Fig. 1c ; Supplementary Fig. S2a , CYLD expression in the lung tissues with fibrosis was much lower compared with that in normal control. We next sought to explore why CYLD protein level is lower in patients with fibrosis. Because TGF-β-expression was found to be upregulated at a later stage of infection during recovery process from tissue injury, we sought to determine whether TGF-β regulates CYLD expression. Indeed, the expression of CYLD was inhibited by TGF-β in the lung tissue of mice ( Supplementary Fig. S2b ). Thus, it is logical to propose that TGF-β may promote tissue fibrosis not only by activating the TGF-β-Smad signalling pathway, the critical positive regulator for fibrotic response, but may also, at least in part, by inhibiting the expression of CYLD, the negative regulator for fibrotic response. How TGF-β regulates CYLD needs to be further investigated in the future studies. To further evaluate the generalizability of our findings, we next sought to determine whether CYLD also acts as a key negative regulator for chemical-induced lung fibrosis in a widely used lung fibrosis model induced by bleomycin. Interestingly, as shown in Supplementary Fig. S3 , bleomycin-induced lung fibrosis was also significantly enhanced in Cyld-deficient mice compared with WT mice. These data thus suggest that the anti-fibrotic effect of CYLD via inhibiting TGF-β-signalling may be generalizable for tissue fibrosis induced by other injurious stimuli as well. CYLD prevents lung fibrosis via inhibiting TGF-β-signalling Because S. pneumoniae induces TGF-β-signalling and TGF-β-signalling is known as a crucial signalling pathway involved in the development of lung fibrosis [10] , [11] , [12] , [13] , [14] , [15] , [16] , we determined whether CYLD inhibits TGF-β-signalling using various approaches including short interfering RNA (siRNA). As expected, siRNA-CYLD (siCYLD) efficiently reduced endogenous CYLD protein expression in a number of cell types including human primary bronchial epithelial NHBE cells and greatly enhanced TNF-α-induced activation of NF-κB-Luc activity, as previously shown ( Fig. 2a,b ). Interestingly, CYLD knockdown with siCYLD markedly enhanced the activity of TGF-β-induced Smad-binding element (SBE)-dependent promoter and TGF-β-responsive PAI-1 promoter activity as well as PAI-1 messenger RNA in human lung epithelial A549 and HeLa cells ( Fig. 2c,d ). Consistent with these results, siCYLD enhanced, whereas overexpressing WT-CYLD, inhibited TGF-β-induced SBE-dependent promoter activity in a dose-dependent manner ( Fig. 2e ). We next confirmed this finding in human primary bronchial epithelial NHBE cells. As shown in Fig. 2f , siCYLD enhanced, whereas overexpressing WT-CYLD inhibited, TGF-β-induced SBE-Luc activity in NHBE cells. Consistent with the results obtained using siCYLD, CYLD deficiency also enhanced TGF-β-induced SBE-Luc activation in Cyld −/− mouse embryonic fibroblast (MEF) cells as compared with WT MEF ( Fig. 2g ). Moreover, CYLD deficiency also markedly enhanced induction of TGF-β-regulated fibrogenic genes in mouse lung tissue, including PAI-1 and CTGF ( Fig. 2h ). We conclude from these data that CYLD negatively regulates TGF-β-signalling both in vitro and in vivo . We further investigated whether CYLD deficiency leads to lung fibrosis via enhancement of TGF-β-signalling by using SB431542, a specific inhibitor of TGF-β-signalling. Indeed, as shown in Fig. 2i , systemic inoculation of SB431542 inhibited lung fibrosis in S. pneumoniae -inoculated Cyld −/− lungs, thereby confirming that CYLD deficiency leads to pulmonary fibrosis in post bacterial infections via enhancing TGF-β-signalling. 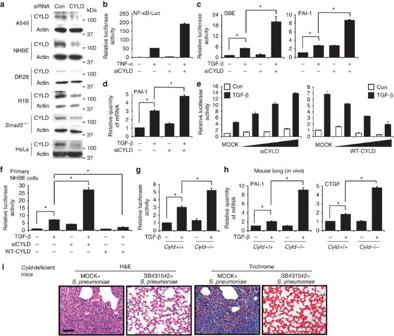Figure 2: CYLD prevents development of lung fibrosis via inhibition of TGF-β-signalling. (a) Epithelial cells transfected with siRNA-Control (siCon) or siCYLD were analysed by immunoblotting with the indicated antibodies. (b) NF-κB-promoter activity was determined in siCon- or siCYLD-transfected cells stimulated with TNF-α (10 ng ml−1). (c) SBE-promoter and PAI-1-promoter activity was determined in siRNA-control (siCon) or siCYLD-transfected cells stimulated with TGF-β. (d) Relative quantity of PAI-1 mRNA expression compared with Glyceraldehyde 3-phosphate dehydrogenase was measured in siCon- or siCYLD-transfected cells stimulated with TGF-β. (e) SBE-promoter activity was determined in A549 cells transfected with various amount of siCYLD or WT-CYLD and stimulated with TGF-β. (f) SBE-promoter activity was determined in siCYLD or WT-CYLD-transfected human primary bronchial epithelial NHBE cells stimulated with TGF-β. (g) SBE-promoter activity was determined in mouse MEFs fromCyld+/+andCyld−/−mice stimulated with TGF-β. (h) Relative quantity of mRNA expression of PAI-1 and CTGF compared with Glyceraldehyde 3-phosphate dehydrogenase was measured in the lung tissues ofCyld+/+andCyld−/−mice 6-h post-i.t. inoculation of TGF-β (25–100 ng per mouse).*P<0.05 values in (b–h) are the means±s.d. (n=3). Statistical data analysis was performed using Student'st-test. (i) H&E and Masson's trichrome staining of lung tissues fromCyld−/−mice 2-weeks post-S. pneumoniae-infection with or without intraperitoneal inoculation of SB431542 (10 mg per kg body weight). Scale bars, 200 μm. Figure 2: CYLD prevents development of lung fibrosis via inhibition of TGF-β-signalling. ( a ) Epithelial cells transfected with siRNA-Control (siCon) or siCYLD were analysed by immunoblotting with the indicated antibodies. ( b ) NF-κB-promoter activity was determined in siCon- or siCYLD-transfected cells stimulated with TNF-α (10 ng ml −1 ). ( c ) SBE-promoter and PAI-1-promoter activity was determined in siRNA-control (siCon) or siCYLD-transfected cells stimulated with TGF-β. ( d ) Relative quantity of PAI-1 mRNA expression compared with Glyceraldehyde 3-phosphate dehydrogenase was measured in siCon- or siCYLD-transfected cells stimulated with TGF-β. ( e ) SBE-promoter activity was determined in A549 cells transfected with various amount of siCYLD or WT-CYLD and stimulated with TGF-β. ( f ) SBE-promoter activity was determined in siCYLD or WT-CYLD-transfected human primary bronchial epithelial NHBE cells stimulated with TGF-β. ( g ) SBE-promoter activity was determined in mouse MEFs from Cyld +/+ and Cyld −/− mice stimulated with TGF-β. ( h ) Relative quantity of mRNA expression of PAI-1 and CTGF compared with Glyceraldehyde 3-phosphate dehydrogenase was measured in the lung tissues of Cyld +/+ and Cyld −/− mice 6-h post-i.t. inoculation of TGF-β (25–100 ng per mouse). *P< 0.05 values in ( b – h ) are the means±s.d. ( n =3). Statistical data analysis was performed using Student's t -test. ( i ) H&E and Masson's trichrome staining of lung tissues from Cyld −/− mice 2-weeks post- S. pneumoniae -infection with or without intraperitoneal inoculation of SB431542 (10 mg per kg body weight). Scale bars, 200 μm. Full size image CYLD inhibits TGF-β-signalling via decreasing Smad3 stability Having identified CYLD as a negative regulator of TGF-β-signalling and lung fibrosis, we next sought to determine how CYLD inhibits TGF-β-signalling. TGF-β-ligands bind to a type II receptor (TβRII), which recruits and phosphorylates a type I receptor (TβRI). The activated TβRI then phosphorylates the Smad subgroup known as receptor-activated Smads (R-Smad), for example, Smad3, which can bind to Co-Smad Smad4. The R-Smad and Co-Smad complex then undergoes nuclear translocation for target gene regulation [17] , [18] , [19] , [20] . To first determine at which level CYLD inhibits TGF-β-signalling, we took advantage of the available lung epithelial cell lines, DR26 and R1B that are derived from the WT Mv1Lu cells and lack functional TβRII and TβRI, respectively [21] . As shown in Fig. 3a , siCYLD markedly enhanced constitutively active (C/A)-TβRI-induced SBE-Luc activity in TβRII-deficient DR26 cells, suggesting enhancement of TGF-β-signalling, by CYLD knockdown, occurs at the level or downstream of TβRI independent of TβRII. We next determined whether CYLD exerts its inhibitory effect on TGF-β-signalling at the level or downstream of TβRI by assessing the effects of siCYLD on WT-Smad3-induced SBE-Luc activity in TβRI-deficient R1B cells. CYLD knockdown markedly enhanced WT-Smad3-induced SBE-Luc activation in R1B cells, suggesting CYLD may inhibit TGF-β-signalling at the level or downstream of Smad3 independent of TβRI ( Fig. 3b ). To further determine whether CYLD inhibits TGF-β-signalling by likely targeting Smad3, we next evaluated the effect of CYLD knockdown in Smad3-deficient MEF cells. As shown in Fig. 3c , siCYLD did not enhance SBE-Luc activity in the absence of Smad3. In contrast, siCYLD markedly enhanced SBE-Luc activity in cells reconstituted with WT-Smad3, suggesting CYLD may inhibit TGF-β-signalling at the level of, or downstream of, Smad3. 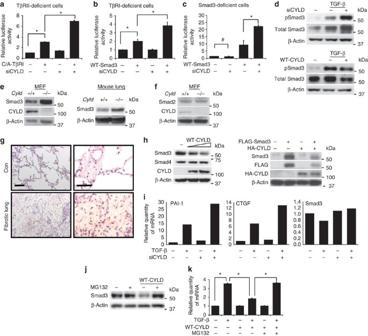Figure 3: CYLD inhibits TGF-β-signalling via decreasing stability of Smad3 protein. (a) SBE-promoter activity was determined in siCon- or siCYLD-transfected TβII-deficient DR26 cells co-transfected with control vector or constitutively active (C/A)-TβRI. (b) SBE-promoter activity was determined in siCON- or siCYLD-transfected TβI-deficient R1B cells co-transfected with control vector or WT-Smad3. (c) SBE-promoter activity was determined in siCON- or siCYLD-transfectedSmad3−/−MEF cells, co-transfected with control vector or WT-Smad3. (d) Cells transfected with siCYLD or WT-CYLD were treated with TGF-β and analysed by immunoblotting with the indicated antibodies. (e,f) MEF cells and lung tissues fromCyld+/+andCyld−/−mice were analysed by immunoblotting with the indicated antibodies. (g) Lung tissues from control (Con) and lung fibrosis patients (Fibrotic lung) were stained against Smad3 (Left panels, ×100; right panels, ×400). Scale bars, 200 μm. (h) Cells transfected with WT-CYLD with (right panel) or without Flag-WT-Smad3 (left panel) were analysed by immunoblotting with the indicated antibodies. (i) Relative quantity of mRNA expressions of PAI-1, CTGF, and Smad3 compared with Glyceraldehyde 3-phosphate dehydrogenase was measured in A549 cells transfected with siCON or siCYLD and stimulated with TGF-β. (j) Cells transfected with control vector or WT-CYLD were treated with MG132 (20 μM) and analysed by immunoblotting with the indicated antibodies. (k) Cells transfected with WT-CYLD were pre-treated with MG-132, and relative quantity of PAI-1 mRNA expression, compared with Glyceraldehyde 3-phosphate dehydrogenase, was measured post-TGF-β-treatment.*P<0.05, #P>0.05 values ina,b,c,i, andkare the means±s.d. (n=3). Statistical data analysis was performed using Student'st-test. Figure 3: CYLD inhibits TGF-β-signalling via decreasing stability of Smad3 protein. ( a ) SBE-promoter activity was determined in siCon- or siCYLD-transfected TβII-deficient DR26 cells co-transfected with control vector or constitutively active (C/A)-TβRI. ( b ) SBE-promoter activity was determined in siCON- or siCYLD-transfected TβI-deficient R1B cells co-transfected with control vector or WT-Smad3. ( c ) SBE-promoter activity was determined in siCON- or siCYLD-transfected Smad3 −/− MEF cells, co-transfected with control vector or WT-Smad3. ( d ) Cells transfected with siCYLD or WT-CYLD were treated with TGF-β and analysed by immunoblotting with the indicated antibodies. ( e,f ) MEF cells and lung tissues from Cyld +/+ and Cyld −/− mice were analysed by immunoblotting with the indicated antibodies. ( g ) Lung tissues from control (Con) and lung fibrosis patients (Fibrotic lung) were stained against Smad3 (Left panels, ×100; right panels, ×400). Scale bars, 200 μm. ( h ) Cells transfected with WT-CYLD with (right panel) or without Flag-WT-Smad3 (left panel) were analysed by immunoblotting with the indicated antibodies. ( i ) Relative quantity of mRNA expressions of PAI-1, CTGF, and Smad3 compared with Glyceraldehyde 3-phosphate dehydrogenase was measured in A549 cells transfected with siCON or siCYLD and stimulated with TGF-β. ( j ) Cells transfected with control vector or WT-CYLD were treated with MG132 (20 μM) and analysed by immunoblotting with the indicated antibodies. ( k ) Cells transfected with WT-CYLD were pre-treated with MG-132, and relative quantity of PAI-1 mRNA expression, compared with Glyceraldehyde 3-phosphate dehydrogenase, was measured post-TGF-β-treatment. *P< 0.05, # P> 0.05 values in a , b , c , i , and k are the means±s.d. ( n =3). Statistical data analysis was performed using Student's t -test. Full size image To further determine how CYLD inhibits TGF-β-signalling via Smad3, we next evaluated the effect of CYLD on Smad3 activation by using antibody against phosphorylated Smad3. Interestingly, CYLD knockdown increased, whereas overexpressing WT-CYLD, inhibited not only phosphorylated but also total Smad3 ( Fig. 3d ). Smad3 expression is also higher in both Cyld −/− MEF and Cyld −/− mouse lung compared with their WT counterparts ( Fig. 3e ), whereas another R-Smad Smad2 expression was unaffected by CYLD deficiency ( Fig. 3f ). Consistent with these results, Smad3 expression was also higher in the lung of human patients with pulmonary fibrosis as compared with normal control ( Fig. 3g; Supplementary Fig. S2a ). Moreover, overexpressing WT-CYLD markedly reduced expression of both endogenous and exogenous Smad3, but not Smad4 proteins ( Fig. 3h ), but had no effect on the levels of Smad3 mRNA ( Fig. 3i ). Interestingly, treatment with MG132, a specific proteasome inhibitor, reversed the WT-CYLD-induced decrease in Smad3 protein level ( Fig. 3j ) and TGF-β-induced PAI-1 expression ( Fig. 3k ). Collectively, these data suggest that CYLD inhibits TGF-β-signalling by decreasing stability of Smad3 protein in a proteasome-dependent manner. CYLD decreases Smad3 stability via Akt-GSK3β-CHIP pathway Because CYLD is a known deubiquitinating enzyme (DUB) [22] , [23] , [24] , [25] , [26] , [27] , [28] , [29] , we investigated whether CYLD-induced Smad3 degradation depends on its deubiquitinating activity. We first assessed the effect of DUB-deficient CYLD mutants on Smad3 basal level and TGF-β-induced SBE promoter activity. As shown in Fig. 4a , DUB-deficient CYLD mutants (H/N-CYLD and C/S-CYLD) failed to induce Smad3 degradation as compared with WT-CYLD. Similar result was also observed in TGF-β-induced SBE promoter activity ( Fig. 4b ). These data suggest that CYLD decreases Smad3 stability in a DUB activity-dependent manner. 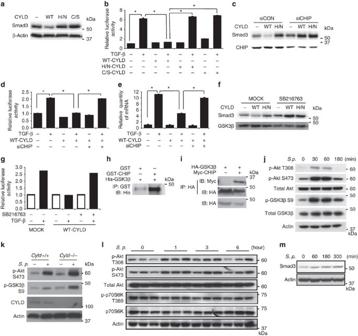Figure 4: CYLD decreases stability of Smad3 protein in a GSK3β-CHIP-dependent manner possibly via Akt. (a) Cells transfected with WT-CYLD or DUB-deficient mutants (H/N-CYLD or C/S-CYLD) were analysed by immunoblotting with the indicated antibodies. (b) SBE-promoter activity was determined in cells transfected with WT-CYLD, H/N-CYLD or C/S-CYLD stimulated with TGF-β. (c) Cells co-transfected with siCon or siCHIP with WT-CYLD or H/N-CYLD were analysed by immunoblotting with the indicated antibodies. (d) SBE-promoter activity was determined in cells co-transfected with siCon or siCHIP with WT-CYLD stimulated with TGF-β. (e) Relative quantity of PAI-1 mRNA expression compared with Glyceraldehyde 3-phosphate dehydrogenase was measured in cells co-transfected with siCon or siCHIP with WT-CYLD stimulated with TGF-β. (f) Cells transfected with control vector, WT-CYLD or DUB-deficient H/N-CYLD were treated with vehicle control or GSK3β-inhibitor SB216763 (5 μM) for 12 h and analysed by immunoblotting with the indicated antibodies. (g) Cells transfected with control vector or WT-CYLD were pre-treated with GSK3β-inhibitor (5 μM) for 2 h, followed by TGF-β-stimulation, and SBE-promoter activity was then determined. (h) Recombinant GSK3β protein (His-GSK3β) was incubated either with GST or recombinant CHIP protein (GST-CHIP)in vitro. CHIP was pulled down with Sepharose 4B beads and immunoblotted against His to detect GSK3β. (i) HA-GSK3β in cells co-transfected with Myc-CHIP and HA-GSK3β was pulled down with HA probe and analysed by immunoblotting with anti-Myc antibody. (j) A549 cells were treated withS. pneumoniaefor various times as indicated in the figure, and cell lysates were analysed by immunoblotting with the indicated antibodies. (k) MEF cells fromCyld+/+andCyld−/−mice were treated withS. pneumoniaefor 30 min, and cell lysates were analysed by immunoblotting with the indicated antibodies. (l) WT mice were i.t. inoculated withS. pneumoniaefor various times as indicated in the figure, and proteins from lung tissues were analysed by immunoblotting with the indicated antibodies. (m) A549 cells were treated withS. pneumoniaefor various times as indicated, and cell lysates were analysed by immunoblotting with the indicated antibodies.*P<0.05 values inb,d,e, andgare the means±s.d. (n=3). Statistical data analysis was performed using Student'st-test.S.p.,Streptococcus pneumonia. Figure 4: CYLD decreases stability of Smad3 protein in a GSK3β-CHIP-dependent manner possibly via Akt. ( a ) Cells transfected with WT-CYLD or DUB-deficient mutants (H/N-CYLD or C/S-CYLD) were analysed by immunoblotting with the indicated antibodies. ( b ) SBE-promoter activity was determined in cells transfected with WT-CYLD, H/N-CYLD or C/S-CYLD stimulated with TGF-β. ( c ) Cells co-transfected with siCon or siCHIP with WT-CYLD or H/N-CYLD were analysed by immunoblotting with the indicated antibodies. ( d ) SBE-promoter activity was determined in cells co-transfected with siCon or siCHIP with WT-CYLD stimulated with TGF-β. ( e ) Relative quantity of PAI-1 mRNA expression compared with Glyceraldehyde 3-phosphate dehydrogenase was measured in cells co-transfected with siCon or siCHIP with WT-CYLD stimulated with TGF-β. ( f ) Cells transfected with control vector, WT-CYLD or DUB-deficient H/N-CYLD were treated with vehicle control or GSK3β-inhibitor SB216763 (5 μM) for 12 h and analysed by immunoblotting with the indicated antibodies. ( g ) Cells transfected with control vector or WT-CYLD were pre-treated with GSK3β-inhibitor (5 μM) for 2 h, followed by TGF-β-stimulation, and SBE-promoter activity was then determined. ( h ) Recombinant GSK3β protein (His-GSK3β) was incubated either with GST or recombinant CHIP protein (GST-CHIP) in vitro . CHIP was pulled down with Sepharose 4B beads and immunoblotted against His to detect GSK3β. ( i ) HA-GSK3β in cells co-transfected with Myc-CHIP and HA-GSK3β was pulled down with HA probe and analysed by immunoblotting with anti-Myc antibody. ( j ) A549 cells were treated with S. pneumoniae for various times as indicated in the figure, and cell lysates were analysed by immunoblotting with the indicated antibodies. ( k ) MEF cells from Cyld +/+ and Cyld −/− mice were treated with S. pneumoniae for 30 min, and cell lysates were analysed by immunoblotting with the indicated antibodies. ( l ) WT mice were i.t. inoculated with S. pneumoniae for various times as indicated in the figure, and proteins from lung tissues were analysed by immunoblotting with the indicated antibodies. ( m ) A549 cells were treated with S. pneumoniae for various times as indicated, and cell lysates were analysed by immunoblotting with the indicated antibodies. *P< 0.05 values in b , d , e , and g are the means±s.d. ( n =3). Statistical data analysis was performed using Student's t -test. S.p. , Streptococcus pneumonia . Full size image Because E3 ubiquitin ligase has a critical role in mediating Smad3 degradation [30] and CYLD is known as a deubiquitinase [22] , [28] , [29] , we hypothesized that CYLD may decrease Smad3 stability via regulating an E3 ubiquitin ligase. On the basis that carboxy terminus of CHIP has been shown to mediate Smad3 degradation [31] , [32] , we first determined whether CHIP mediates CYLD-induced Smad3 degradation by using siCHIP. The efficiency of siCHIP in reducing CHIP expression was first confirmed in A549 cells ( Supplementary Fig. S4 ). As shown in Fig. 4c , CHIP knockdown using siCHIP reversed the WT-CYLD-induced Smad3 decrease in A549 cells. Similar results were also observed in TGF-β-induced SBE promoter activity and PAI-1 upregulation ( Fig. 4d,e , respectively). We next examined whether CYLD directly interacts with CHIP by performing co-immunoprecipitation experiments. As shown in Supplementary Fig. S5 , no direct physical interaction was observed between CYLD and CHIP, thereby suggesting that CYLD may regulate CHIP-dependent Smad3 stability probably by targeting an upstream molecule of CHIP. In view of the known upstream signalling, molecules involved in mediating Smad3 degradation, GSK3β was shown to have an important role in mediating Smad3 degradation [33] . We thus determined whether GSK3β is involved in mediating CYLD-induced Smad3 degradation. As shown in Fig. 4f , a specific GSK3β inhibitor SB216763 reversed the WT-CYLD-induced Smad3 decrease in A549 cells. Similar results were also observed in TGF-β-induced SBE promoter activity ( Fig. 4g ), thereby suggesting the involvement of GSK3β in mediating regulation of Smad3 stability by CYLD. We further performed co-immunoprecipitation experiments to determine whether GSK3β directly interacts with CYLD. As shown in Supplementary Fig. S5 , no direct interaction was found between GSK3β and CYLD, suggesting the involvement of an additional signalling molecule, further upstream of GSK3β. It is interesting to note that GSK3β was found to directly interact with CHIP both in vitro and in vivo ( Fig. 4h,i ). Further experiments demonstrate that GSK3β phosphorylation was induced by S. pneumoniae and enhanced by CYLD deficiency ( Fig. 4j,k ). As phosphorylation of GSK3β is known to result in inactivation of its kinase activity and CYLD deficiency enhances GSK3β phosphorylation, it is logical that CYLD may induce GSK3β kinase activity by inhibiting its phosphorylation and thereby promoting GSK3β-CHIP-mediated Smad3 protein degradation. However, it still remains unclear how GSK3β regulates CHIP-mediated Smad3 protein degradation. Previously, it has been reported that Erk5 MAPK regulates E3 ligase activity of CHIP dependently on Erk5 kinase activity [34] . Thus, it is likely that GSK3β may regulate E3 ligase activity of CHIP by binding to CHIP dependently on GSK3β kinase activity. Further investigation is needed for understanding the molecular mechanism underlying GSK3β-mediated regulation of CHIP E3 ligase activity. We next sought to determine the direct molecular target of CYLD in mediating GSK3β-dependent Smad3 protein degradation. Because Akt is known as the major upstream regulator of GSK3β [35] , [36] , we investigated whether Akt mediates CYLD-induced degradation of Smad3. We first determined whether S. pneumoniae induces activation of Akt. As shown in Fig. 4j–l , S . pneumoniae induced phosphorylation of Akt and GSK3β, but not p70S6K, which represents another downstream target of PI3K pathway, suggesting the specific activation of Akt-GSK3β by S. pneumoniae. Consistent with these results, S. pneumoniae also upregulated Smad3 protein expression in a time-dependent manner ( Fig. 4m ). This interesting result thus led us to determine whether Akt is critically involved in mediating CYLD-induced degradation of Smad3 by first examining the effect of Akt knockdown on Smad3 protein stability. CYLD decreases Smad3 stability by inhibiting Akt As shown in Supplementary Fig. S6a , Akt1 and 2 but not 3 are predominantly expressed in both Cyld +/+ and Cyld −/− cells. Thus, we determined the effect of knockdown of both Akt1 and 2 on Smad3 protein level in these cells. As shown in Fig. 5a , knockdown of Akt1/2 significantly reduced Smad3 protein expression in both WT and Cyld-deficient cells. Consistent with this result, Akt knockdown also inhibited the enhancement of TGF-β-induced SBE promoter activity induced by CYLD knockdown ( Fig. 5b ). Similarly, enhanced TGF-β-induced SBE promoter activity was also inhibited by Akt-specific inhibitor in Cyld −/− MEFs ( Fig. 5c ). Moreover, TGF-β-induced PAI-1 mRNA expression was also markedly reduced by Akt1-deficiency in Akt1 −/− cells, and siCYLD no longer enhanced TGF-β-induced PAI-1 expression in Akt1 −/− cells ( Supplementary Fig. S6b ). We further confirmed whether activation of Akt does induce upregulation of fibrotic response gene expression via Smad3. As shown in Supplementary Fig. S7 , activation of Akt by expressing a constitutively active C/A-Akt indeed induced expression of PAI-1 and CTGF in Smad3 +/+ cells, but not in Smad3 −/− cells. Together, these data provide supportive evidence for the critical involvement of Akt in mediating CYLD-dependent Smad3 degradation. PI3 K is known as the one of the major signalling molecules upstream of Akt. We thus determined whether PI3K, like Akt, is also involved in mediating CYLD-dependent Smad3 degradation by evaluating the effect of PI3K and Akt inhibitors on Smad3 protein expression. Akt inhibitor markedly reduced Smad3 protein expression whereas PI3K inhibitor LY294002 did not reduce Smad3 protein expression ( Fig. 5d,e ). These results are rather unexpected as it is well known that PI3K and, in turn, PIP3 is completely rate-limiting for Akt activation [37] . Because only chemical inhibitors for PI3K were used in our studies, our data do not completely preclude the possible involvement of PI3K in regulating Akt-mediated regulation of Smad3. Further studies are needed to determine whether CYLD-Akt-mediated regulation of Smad3 is indeed independent of PI3K by using more specific approaches. Nonetheless, these data suggest that CYLD decreases Smad3 protein stability via negatively regulating Akt. 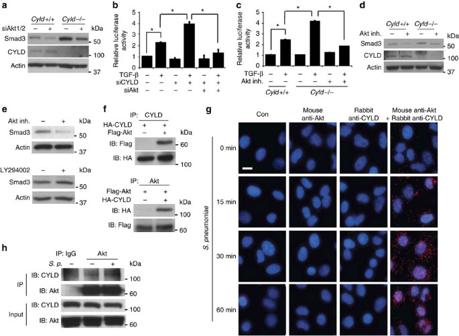Figure 5: CYLD decreases Smad3 stability by inhibiting Akt. (a) MEF cells fromCyld+/+andCyld−/−mice were transfected with siCon or siAkt1/2 and analysed by immunoblotting with the indicated antibodies. (b) SBE-promoter activity was determined in siCYLD-transfected A549 cells with or without siAkt co-transfection and stimulated with TGF-β. (c) SBE-promoter activity was determined in MEFs fromCyld+/+andCyld−/−mice pretreated with Akt inhibitor and stimulated with TGF-β. (d) MEF cells fromCyld+/+andCyld−/−mice were incubated with Akt inhibitor (20 μM), and cell lysates were analysed by immunoblotting with the indicated antibodies. (e) Cells were incubated with Akt inhibitor (20 μM) or LY294002 (20 μM), and cell lysates were analysed by immunoblotting with the indicated antibodies. (f) Lysates from cells transfected with HA-CYLD and Flag-Akt were immunoprecipitated with anti-CYLD antibody (upper panel) or anti-Akt antibody (lower panel), and interacting proteins were analysed by immunoblotting. (g) A549 cells were treated withS. pneumoniaefor various times as indicated in the figure, stained with rabbit anti-CYLD antibody and/or mouse anti-Akt antibody, andin vivoprotein–protein interaction between CYLD, and Akt (Red dot) was detected with secondary proximity probes, anti-Rabbit MINUS and anti-mouse-PLUS, using Duolinkin vivoprotein–protein interaction detection kit (Olink). Scale bar, 10 μm. (h) Cells were treated withS. pneumoniaeor vehicle control. Akt in cell lysates was pulled down with anti-Akt antibody and immunoblotted against CYLD and Akt.*P<0.05 values inb,care the means±s.d. (n=3). Statistical data analysis was performed using Student'st-test.S.p.,Streptococcus pneumonia. Figure 5: CYLD decreases Smad3 stability by inhibiting Akt. ( a ) MEF cells from Cyld +/+ and Cyld −/− mice were transfected with siCon or siAkt1/2 and analysed by immunoblotting with the indicated antibodies. ( b ) SBE-promoter activity was determined in siCYLD-transfected A549 cells with or without siAkt co-transfection and stimulated with TGF-β. ( c ) SBE-promoter activity was determined in MEFs from Cyld +/+ and Cyld −/− mice pretreated with Akt inhibitor and stimulated with TGF-β. ( d ) MEF cells from Cyld +/+ and Cyld −/− mice were incubated with Akt inhibitor (20 μM), and cell lysates were analysed by immunoblotting with the indicated antibodies. ( e ) Cells were incubated with Akt inhibitor (20 μM) or LY294002 (20 μM), and cell lysates were analysed by immunoblotting with the indicated antibodies. ( f ) Lysates from cells transfected with HA-CYLD and Flag-Akt were immunoprecipitated with anti-CYLD antibody (upper panel) or anti-Akt antibody (lower panel), and interacting proteins were analysed by immunoblotting. ( g ) A549 cells were treated with S. pneumoniae for various times as indicated in the figure, stained with rabbit anti-CYLD antibody and/or mouse anti-Akt antibody, and in vivo protein–protein interaction between CYLD, and Akt (Red dot) was detected with secondary proximity probes, anti-Rabbit MINUS and anti-mouse-PLUS, using Duolink in vivo protein–protein interaction detection kit (Olink). Scale bar, 10 μm. ( h ) Cells were treated with S. pneumoniae or vehicle control. Akt in cell lysates was pulled down with anti-Akt antibody and immunoblotted against CYLD and Akt. *P< 0.05 values in b , c are the means±s.d. ( n =3). Statistical data analysis was performed using Student's t -test. S.p. , Streptococcus pneumonia . Full size image To further determine how CYLD negatively regulates Akt, we first examined whether CYLD physically interacts with Akt by performing co-immunoprecipitation experiments. Results in Fig. 5f showed that CYLD and Akt are indeed physically associated with each other in epithelial cells co-transfected with HA-CYLD and Flag-Akt. We next determined whether endogenous CYLD directly interacts with endogenous Akt and if such a direct interaction is further increased on S. pneumoniae treatment by performing Duolink in vivo protein–protein interaction detection assay [38] , [39] and co-immunoprecipitation assay. As shown in Fig. 5g,h , endogenous CYLD indeed directly interacts with endogenous Akt and S. pneumoniae treatment increased their direct interaction. Together, these data suggest that CYLD decreases Smad3 stability and TGF-β-signalling by inhibiting Akt. CYLD deubiquitinates K63-ubiquitinated Akt to inhibit Smad3 Because CYLD is a known deubiquitinase and Akt ubiquitination is critical for its functional activity [40] , we next investigated whether CYLD deubiquitinates Akt. As shown in Fig. 6a , co-expressing WT-CYLD, but not DUB mutant (H/N-CYLD), decreased Akt polyubiquitination. In addition, siCYLD also markedly enhanced S. pneumoniae -induced Akt ubiquitination in epithelial cells ( Fig. 6b ). We then determined whether S. pneumoniae induces endogenous Akt ubiquitination in the absence and presence of CYLD. As shown in Fig. 6c,d ; Supplementary Fig. S8 , endogenous Akt ubiquitination was detected in the absence of S. pneumoniae , and S. pneumoniae markedly enhanced endogenous Akt ubiquitination. Interestingly, expression of WT-CYLD greatly decreased S. pneumoniae -induced endogenous Akt ubiquitination, whereas CYLD knockdown, or CYLD deficiency, enhanced it. Because Akt has been shown to undergo K63 polyubiquitination, we next determined whether CYLD specifically deubiquitinates K63-polyubiquitinated Akt. As shown in Fig. 6e , co-expressing WT-CYLD markedly decreased K63- but not K48-polyubiquitinated Akt. Consistently, results in Fig. 6f indicate that recombinant CYLD protein (GST-rCYLD) directly deubiquitinates K63-linked polyubiquitination of Akt (His-rAkt) in vitro in a cell-free system in a dose-dependent manner. Moreover, deficiency of CYLD also enhanced S. pneumoniae -induced K63-polyubiquitination of Akt ( Fig. 6g ). Taken together, these data provide strong evidence that CYLD negatively regulates Akt by directly interacting with and deubiquitinating K63-polyubiquitinated Akt, both in vitro in a cell-free system and in vivo under endogenous condition. 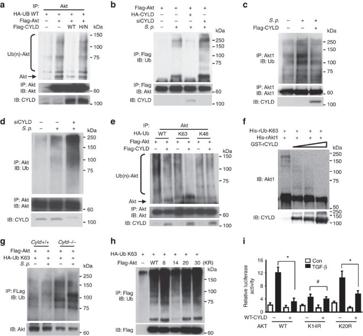Figure 6: CYLD deubiquitinates K63-polyubiquitinated Akt to reduce Smad3. (a) Lysates from A549 cells co-transfected with HA-Ub WT, Flag-Akt WT, Flag-WT-CYLD or Flag-H/N-CYLD were immunoprecipitated with anti-Akt antibody and analysed by immunoblotting with the indicated antibodies. (b) Cells were co-transfected with Flag-Akt, HA-CYLD, or siCYLD and treated withS. pneumoniae. Akt was pulled down with Flag probe and immunoblotted against Ubiquitin (Ub), Akt, and CYLD. (c) Cells transfected with control vector or Flag-WT-CYLD were treated withS. pneumoniae, and cell lysates were immunoprecipitated with anti-Akt1 antibody and analysed by immunoblotting with the indicated antibodies. (d) CYLD-depleted cells using siCYLD were treated withS. pneumoniae, and Akt in cell lysates was pulled down with anti-Akt antibody and immunoblotted against Ub, Akt, and CYLD. (e) Lysates from A549 cells co-transfected with Flag-Akt WT, Flag-WT-CYLD, HA-Ub WT, HA-Ub K63, or HA-Ub K48 were immunoprecipitated with anti-Akt antibody, and analysed by immunoblotting with the indicated antibodies. (f) Recombinant Akt1 (His-rAkt1) was incubated with recombinant K63 ubiquitin (His-rUb-K63) with or without recombinant CYLD (GST-rCYLD) inin vitroubiquitination assay buffer (BostonBiochem) and analysed by immunoblotting with the indicated antibodies. (g) MEF cells fromCyld+/+andCyld−/−mice were co-transfected with Flag-Akt and HA-Ub K63, and treated withS. pneumoniae. Akt in cell lysate was pulled down with Flag probe and immunoblotted against Ub and Akt. (h) Lysates from cells co-transfected with HA-Ub K63, Flag-Akt WT, or Flag-Akt KR mutants (K8R, K14R, K20R or K30R) were immunoprecipitated with anti-Flag probe and analysed by immunoblotting with the indicated antibodies. (i) SBE-promoter activity was determined in A549 cells co-transfected with WT-CYLD, Akt WT, Akt K14R or Akt K20R stimulated with TGF-β.*P<0.05, #P>0.05 values iniare the means±s.d. (n=3). Statistical data analysis was performed using Student'st-test.S.p.,Streptococcus pneumonia. Figure 6: CYLD deubiquitinates K63-polyubiquitinated Akt to reduce Smad3. ( a ) Lysates from A549 cells co-transfected with HA-Ub WT, Flag-Akt WT, Flag-WT-CYLD or Flag-H/N-CYLD were immunoprecipitated with anti-Akt antibody and analysed by immunoblotting with the indicated antibodies. ( b ) Cells were co-transfected with Flag-Akt, HA-CYLD, or siCYLD and treated with S. pneumoniae . Akt was pulled down with Flag probe and immunoblotted against Ubiquitin (Ub), Akt, and CYLD. ( c ) Cells transfected with control vector or Flag-WT-CYLD were treated with S. pneumoniae , and cell lysates were immunoprecipitated with anti-Akt1 antibody and analysed by immunoblotting with the indicated antibodies. ( d ) CYLD-depleted cells using siCYLD were treated with S. pneumoniae , and Akt in cell lysates was pulled down with anti-Akt antibody and immunoblotted against Ub, Akt, and CYLD. ( e ) Lysates from A549 cells co-transfected with Flag-Akt WT, Flag-WT-CYLD, HA-Ub WT, HA-Ub K63, or HA-Ub K48 were immunoprecipitated with anti-Akt antibody, and analysed by immunoblotting with the indicated antibodies. ( f ) Recombinant Akt1 (His-rAkt1) was incubated with recombinant K63 ubiquitin (His-rUb-K63) with or without recombinant CYLD (GST-rCYLD) in in vitro ubiquitination assay buffer (BostonBiochem) and analysed by immunoblotting with the indicated antibodies. ( g ) MEF cells from Cyld +/+ and Cyld −/− mice were co-transfected with Flag-Akt and HA-Ub K63, and treated with S. pneumoniae . Akt in cell lysate was pulled down with Flag probe and immunoblotted against Ub and Akt. ( h ) Lysates from cells co-transfected with HA-Ub K63, Flag-Akt WT, or Flag-Akt KR mutants (K8R, K14R, K20R or K30R) were immunoprecipitated with anti-Flag probe and analysed by immunoblotting with the indicated antibodies. ( i ) SBE-promoter activity was determined in A549 cells co-transfected with WT-CYLD, Akt WT, Akt K14R or Akt K20R stimulated with TGF-β. *P< 0.05, # P> 0.05 values in i are the means±s.d. ( n =3). Statistical data analysis was performed using Student's t -test. S.p. , Streptococcus pneumonia . Full size image Because K14 lysine in the pleckstrin homology domain of Akt is critical for mediating its function [40] , we next determined whether mutation of K14 lysine to arginine (R) reduces polyubiquitination of Akt. Indeed, K14R, but not K8R, K20R and K30R, markedly reduced K63-linked polyubiquitination of Akt compared with WT-Akt ( Fig. 6h ). We further determined whether K14 residue in Akt is indeed functionally critical for mediating CYLD-induced inhibition of TGF-β-signalling. As shown in Fig. 6i , expressing WT-CYLD significantly inhibited TGF-β-induced SBE promoter activity in epithelial cells co-transfected with WT-Akt or K20R, but not with K14R, thereby demonstrating the critical role for K14 in the PH domain of Akt in mediating inhibition of TGF-β-signalling by CYLD. TNF receptor-associated factor 6 (TRAF6) was previously shown to function as an E3 ligase for Akt-K63 polyubiquitination and CYLD deubiquitinates TRAF6 (refs 24 , 40 ). Thus, we next explored the possibility that CYLD may inhibit Akt-mediated fibrotic response via deubiquitinating TRAF6. As shown in Supplementary Fig. S9 , CYLD knockdown, using siCYLD, still enhanced TGF-β-induced fibrotic response in TRAF6-depleted cells, thereby suggesting that CYLD inhibits Akt-mediated fibrotic response at least in part by directly interacting with and deubiquitinating Akt. To prevent the development of lung fibrosis during recovery of lung injury, wound-healing responses must be tightly regulated [1] , [4] , [5] , [6] . The molecular mechanisms underlying this tight regulation remain largely unknown. In the present study, we provide evidences to identify CYLD deubiquitinase as a critical negative regulator for preventing development of lung fibrosis after infection with S. pneumoniae . CYLD inhibits TGF-β-signalling and thereby prevents fibrosis via decreasing stability of Smad3 protein in a GSK3β-CHIP-dependent manner. Moreover, CYLD decreases Smad3 protein stability by directly deubiquitinating K63-polyubiquitinated Akt, which, in turn, leads to activation of GSK3β ( Fig. 7a ). CYLD deficiency results in enhanced fibrotic response via enhanced Smad3-protein stability following lung injury ( Fig. 7b ). Taken together, as shown in our previous study [1] , CYLD promotes bacteria-induced lung injury and reduces host survival by inhibiting S. pneumoniae -induced PAI-1 expression via specific inhibition of p38 signalling during early lung-injury stage of infection; and as shown in our current study, CYLD prevents the development of lung fibrosis by inhibiting TGF-β-Smad signalling via reducing Smad3 stability during late tissue remodelling stage of infection. Thus, CYLD acts a key regulator during the entire wound-healing process in lung injury [1] , [41] . These studies may help develop new therapeutic strategy for preventing lung fibrosis. 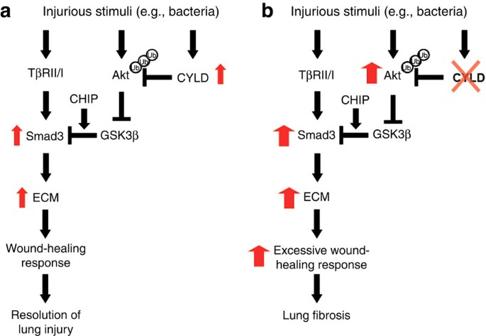Figure 7: A schematic model illustrating a critical role of CYLD in lung fibrosis. (a,b) On the one hand, following lung injury after severe bacterial infection, for example,S. pneumoniaeinfection, extracellular matrix production and tissue recovery process are initiated via both TβRII/I-mediated activation of Smad3 and Akt-dependent inhibition of GSK3β-CHIP-mediated Smad3 degradation. On the other hand, CYLD induced byS. pneumoniaeinhibits Akt by deubiquitinating K63-polyubiquitinated Akt., which in turn leads to activation of GSK3β and promotes CHIP-mediated Smad3 degradation, thereby attenuating excessive fibrotic response and preventing lung fibrosis (a). Deficiency of Cyld results in enhanced activation of Akt, which in turn leads to inhibition of GSK3β and CHIP-mediated Smad3 degradation, thereby promoting excessive fibrotic response and tissue fibrosis (b). ECM, extracellular matrix; TβRII/I, TGF-β receptor II and I. Figure 7: A schematic model illustrating a critical role of CYLD in lung fibrosis. ( a , b ) On the one hand, following lung injury after severe bacterial infection, for example, S. pneumoniae infection, extracellular matrix production and tissue recovery process are initiated via both TβRII/I-mediated activation of Smad3 and Akt-dependent inhibition of GSK3β-CHIP-mediated Smad3 degradation. On the other hand, CYLD induced by S. pneumoniae inhibits Akt by deubiquitinating K63-polyubiquitinated Akt., which in turn leads to activation of GSK3β and promotes CHIP-mediated Smad3 degradation, thereby attenuating excessive fibrotic response and preventing lung fibrosis ( a ). Deficiency of Cyld results in enhanced activation of Akt, which in turn leads to inhibition of GSK3β and CHIP-mediated Smad3 degradation, thereby promoting excessive fibrotic response and tissue fibrosis ( b ). ECM, extracellular matrix; TβRII/I, TGF-β receptor II and I. Full size image Previously it has been known that TNF receptor-associated factor 6 (TRAF6) acts as an E3 ligase for Akt-K63 polyubiquitination, and CYLD deubiquitinates TRAF6 (refs 24 , 40 ). In this study we provided experimental evidences for direct interaction between Akt and CYLD, and also showed that CYLD does directly deubiquitinate Akt under both endogenous and exogenous conditions. It is possible that CYLD may inhibit Akt-mediated fibrotic response by actually deubiquitinating TRAF6. Thus, we evaluated the effect of siCYLD on TGF-β-induced fibrotic response in TRAF6-depleted cells using siTRAF6. Interestingly, CYLD knockdown still led to the enhancement of TGF-β-induced fibrotic response in TRAF6-depleted cells ( Supplementary Fig. S9 ). Nonetheless, these data demonstrate that CYLD indeed inhibits Akt-mediated fibrotic response by at least in part directly interacting with and deubiquitinating Akt. Here we have provided strong evidence that CYLD inhibits S. pneumoniae -induced Smad3-dependent fibrosis via inhibiting Akt, thereby linking CYLD to Smad3 via Akt. It is still unclear whether or not direct activation of Akt induces fibrotic response via Smad3. Indeed, direct activation of Akt by expressing a constitutively active form of C/A-Akt induces expression of fibrotic response gene PAI-1 and CTGF in Smad3 +/+ cells, but not in Smad3 −/− cells ( Supplementary Fig. S7 ). Collectively, it is evident that the fibrotic effects of CYLD-dependent Akt deubiquitination are indeed specifically mediated via the TGF-β-Smad3 pathway. On the basis of the experimental data we presented, it is clear that CYLD regulates lung fibrosis by inhibiting TGF-β-signalling in wound-healing response in lung injury caused by infectious agents. Because TGF-β-signalling has an essential role in regulating tissue fibrotic response, it is possible that CYLD may also be crucial for negatively regulating fibrotic response induced by other injurious stimuli such as caustic chemicals. Thus, we sought to determine whether CYLD also acts as a key negative regulator for chemical-induced lung fibrosis in a widely used lung fibrosis model induced by bleomycin. Interestingly, CYLD deficiency markedly enhanced bleomycin-induced lung fibrosis in Cyld-deficient mice ( Supplementary Fig. S3 ). These data thus suggest that the inhibitory effect of CYLD in fibrotic response may be generalizable for tissue fibrosis induced not only by infectious agents but also by other injurious stimuli such as caustic chemicals, as long as the fibrotic response is mainly mediated via TGF-β-Smad signalling. Cell culture and reagents A549, HeLa and HEK293 cells were maintained in the F12-K, minimal essential medium Eagle's with Earle's balanced salt solution (EMEM), and DMEM, respectively. WT mink Mv1Lu cells and two mutant cell lines DR26 and R1B cells were maintained with EMEM supplemented with nonessential amino acids. MEFs from Smad3 −/− , Cyld +/+ and Cyld −/− mice were maintained in DMEM. Human primary bronchial epithelial NHBE (Cambrex) cells were maintained in bronchial epithelial growth media supplemented with bronchial epithelial growth media single Quot [1] , [24] , [42] , [43] . Recombinant TGF-β1 (indicated as TGF-β throughout the manuscript) and TNF-α were purchased from R&D system; Akt inhibitor (1L6-Hydroxymethyl-chiro-inositol-2(R)-2-O-methyl-3-O-octadecyl-sn-glycerocarbonate) [44] , [45] and SB203580 were from Calbiochem; SB431542 and bleomycin were from Sigma; MG132 was from American Peptide. In vitro ubiquitination and deubiquitination assay kit was purchased from Boston Biochem. Duolink in vivo protein–protein interaction detection assay kit was from Olink Bioscience [38] , [39] . Recombinant His-Akt and His-GSK3β were from Calbiochem. ELISA assay kits for TGF-β and total and phospho-p38 MAPK were purchased from R&D system and Invitrogen, respectively. Real-time quantitative RT–PCR analysis Total RNA was isolated using TRIzol reagent following manufacturer's instructions. Synthesis of complementary DNA from total RNA was performed with MultiScribe reverse transcriptase. Real-time quantitative PCR was performed using an ABI 7500 Sequence Detection System (Applied Biosystems) [24] . Relative quantities of mRNAs were calculated using the comparative threshold cycle method and normalized using human and mouse glyceraldehyde-3-phosphate dehydrogenase as an endogenous control. The primer sequences for mouse COL1A2, COL3A1, CTGF and PAI-1, and human PAI-1, CHIP, and Smad3 are as follows [10] , [11] , [12] . Mouse CTGF: 5′-GTAACCGGGGAGGGAAATTA-3′ and 5′-ACAGCTGGACTCAGCCTCAT-3′; mouse COL1A2: 5′-GACAAATGAATGGGGCAAG-3′ and 5′-CAATGTCCAGAGGTGCAATG-3′; mouse COL3A1: 5′-CGAAGATGGCAAAGATGGAT-3′ and 5′-GCCACTAGGACCCCTTTCTC-3′; mouse PAI-1: 5′-GTAGCACAGGCACTGCAAAA-3′ and 5′-TGAGATGACAAAGGCTGTGG-3′; human PAI-1: 5′-CCCTTTGCAGGATGGAACTA-3′ and 5′-ATGGCAATGTGACTGGAACA-3′; human CHIP: 5′-CCCGGCCCCTATACATAGTT-3′ and 5′-CAGTCCAGAGTCCAACAGCA-3′. Plasmids and luciferase assays The expression plasmids Flag-WT-CYLD, HA-WT-CYLD, Flag-H/N-CYLD, HA-C/S-CYLD, Flag-WT-Smad3, C/A-TβRI, and the reporter plasmids SBE-Luc, PAI-1-Luc, and NF-κB-Luc were previously described [17] , [42] , [43] , [46] . Flag-WT-Akt1, pRK5-HA-Ub WT, pRK5-HA-Ub K63, and pRK5-HA-Ub K48 were from Addgene, and K to R mutants of Akt were generated with WT-Akt1 using QuickChange XL Site-Directed Mutagenesis kit (Stratagene). All transient transfections were carried out using TransIT-LT1 reagent (Mirus) or Lipofectamine (Invitrogen) according to manufacturers' instructions [24] . RNA-mediated interference RNA-mediated Interference for downregulating CYLD expression was carried out using pSuper-CYLD [24] and the sequence for the siCYLD is 5′-GATCCCCGAGCTACTGAGGACAGAAATTCAAGAGATTTCTGTCCTCAGTAG CTCTTTTTGGAAA-3′. Human and mouse siRNAs for Akt and CHIP were from Dharmacon, and knockdown of Akts and CHIP, using siAkt and siCHIP, was performed with Lipofectamine 2000 (Invitrogen). ON-TARGETplus SMARTpool of siRNAs targeting human Akt1, human CHIP, mouse Akt1, and mouse Akt2 consists of four siRNAs and sequences for the siRNAs are as follows: Human siAkt1 (5′-CAUCACACCACCUGACCAA-3′, 5′-ACAAGGACGGGCACAUUAA-3′, 5′-CAAGGGCACUUUCGGCAAG-3′, 5′-UCACAGCCCUGAAGUACUC-3′); human CHIP (5′-CGCUGGUGGCCGUGUAUUA-3′, 5′-GUGGAGGACUACUGAGGUU-3′, 5′-GAAGGAGGUUAUUGACGCA-3′, 5′-UGGAAGAGUGCCAGCGAAA-3′); mouse Akt1 (5′- CUGCAGAACUCUAGGCAUC-3′, 5′-GAUCAAGGAUGGUGCCACU-3′, 5′-GAGGUUGCCCACACGCUUA-3′, 5′-CGACGUAGCCAUUGUGAAG-3′); mouse Akt2 (5′- CCAUGAAUGACUUCGAUUA-3′, 5′-GUACUUUGAUGACGAGUUC-3′, 5′-CCUGAACAAUUUCUCUGUA-3′, 5′-GAUGCGGGCUAUCCAGAUG-3′). Western blot and ubiquitination experiments Western blot, immunoprecipitation and ubiquitination experiments were performed as follows [24] . Western blots were performed using whole-cell extracts, separated on 8 or 10% SDS–PAGE gels, and transferred to polyvinylidine difluoride membranes. The membrane was blocked with a solution of PBS containing 0.1% Tween 20 (PBS-T) and 5% BSA. The membrane was then incubated in a 1:2,000 dilution of a primary antibody in 5% BSA–PBS-T. After three washes in PBS-T, the membrane was incubated with 1:5,000 dilution of the corresponding secondary antibody in 3% non-fact skim milk–PBS-T. Respective proteins were visualized by using enhanced chemiluminescence detection reagents, according to the manufacturer's instructions. To conduct immunoprecipitation analysis, cell lysates were incubated with 1 μg of primary antibodies overnight, at 4 °C, followed by 2-h incubation with protein A/G-agarose beads (Invitrogen). Immnoprecipitates were then suspended in a sample buffer, separated on 8% SDS–PAGE, transferred to polyvinylidine difluoride membrane, and detected by immunoblot analysis, as described above. The antibodies against total-Akt, phospho-Akt at T308 & S473, total Smad3, phospho-Smad3, total p70S6K, phospho-p70S6K at T389, total GSK3β, phospho-GSK3β at S9, mouse HA-Tag, His-Tag, and mouse and rabbit anti-Ubiquitin were purchased from Cell Signaling; antibodies against CYLD, total-Akt1/2/3, goat total-Akt1, Smad4, rabbit HA-Tag, mouse Ubiquitin, and actin were from Santa Cruz; FLAG and β-actin were from Sigma. In vivo protein–protein interaction detection assay A549 cells were cultured in tissue culture slide and incubated with S. pneumoniae , or control for time indicated in the figure. Cells were stained with 2 μg ml −1 of primary mouse anti-Akt antibody and rabbit anti-CYLD antibody, and protein–protein interaction between Akt and CYLD was detected with secondary proximity probes, anti-Rabbit MINUS and anti-mouse PLUS, using Duolink in vivo protein–protein interaction detection assay kit, according to the manufacturer's instructions (Duolink proximity ligation assay, Olink Bioscience) [38] , [39] . Mice and animal experiments Cyld −/− mice were generated by homologous recombination as follows [1] . The targeting construct was designed to disrupt the exons 2 and 3 with an IRES-LacZ/MC1-Neo cassette. The targeting plasmid was linearized and transfected into embryonic stem cells of a 129/S. Homologously recombined embryonic stem cells were injected into blastocysts that were subsequently transferred to foster mothers, to generate chimeric progeny. Generated chimeric progeny were backcrossed to C57BL/6J, and germline transmission was confirmed by PCR with tail DNA. Homozygous knockout of Cyld gene was confirmed by mRNA detection by RT–PCR and CYLD protein detection by western blot analysis in MEF cells and lung tissues. For S. pneumoniae -induced severe infections in WT and Cyld −/− mice, anaesthetized mice were intratracheally (i.t.) inoculated with live S. pneumoniae (5×10 7 CFU per mouse). Survived mice from severe pneumonia were then sacrificed 2 weeks post S. pneumoniae infection for histopathological analysis. For TGF-β inoculation, anaesthetized WT and Cyld −/− mice were i.t. inoculated with TGF-β (25–100 ng per mouse) for 6 h, and lung tissues were then subjected to total mRNA and protein extraction. In experiments using chemical inhibitor, SB431542 (10 mg kg −1 ) or SB203580 (20 mg kg −1 ) or equal volume of vehicle control was administered via an intraperitoneal route 1–2 h(s) before the i.t. inoculation of S. pneumoniae . For bleomycin-induced fibrosis model, animals were i.t. inoculated with bleomycin (3 units per kg body weight) for 2 weeks. Lung tissues were then subjected to histological analysis and total mRNA and protein extraction. All animal experiments were approved by the Institutional Animal Care and Use Committee (IACUC) at University of Rochester and Georgia State University. Histology and immunohistochemistry Lung tissue sections from WT and Cyld −/− mice and normal control and pulmonary fibrosis patients were stained with haematoxylin and eosin (H&E), to visualize lung inflammation, and Masson's trichrome staining (Trichrome staining) was performed to highlight organizing fibrosis. Immunohistochemical staining against CYLD and Smad3 was performed using ABC staining System (Santa Cruz). Briefly, tissue sections were incubated with 1 μg of primary antibodies or control IgG followed by 3 washes with PBS. Tissues were then incubated with 1 μg of biotinylated secondary antibodies followed by the incubation with AB enzyme reagent. After three washes, colour reaction was developed with peroxidase substrate. Control and fibrotic lung tissues from patients were obtained from Chonnam National Hospital with approval from the Institutional Review Board (IRB) at Chonnam National University, Korea. Statistical analysis All experiments were repeated at least three times with consistent results. Data are means±s.d. Statistical significance was assessed by two-tailed unpaired student's t -test. P <0.05 was considered significant. How to cite this article: Lim, J. H. et al . CYLD negatively regulates transforming growth factor-β-signalling via deubiquitinating Akt. Nat. Commun. 3:771 doi: 10.1038/ncomms1776 (2012).